Photoinduced handedness switching in terahertz chiral metamolecules Switching the handedness, or the chirality, of a molecule is of great importance in chemistry and biology, as molecules of different handedness exhibit dramatically different physiological properties and pharmacological effects. Here we experimentally demonstrate handedness switching in metamaterials, a new class of custom-designed composites with deep subwavelength building blocks, in response to external optical stimuli. The metamolecule monolayer flips the ellipticity and rotates the polarization angle of light in excess of 10° under optical excitation, a much stronger electromagnetic effect than that of naturally available molecules. Furthermore, the experimentally demonstrated optical switching effect does not require a structural reconfiguration, which is typically involved in molecular chirality switching and is inherently slow. The handedness switching in chiral metamolecules allows electromagnetic control of the polarization of light and will find important applications in manipulation of terahertz waves, such as dynamically tunable terahertz circular polarizers and polarization modulators for terahertz radiations. Chirality, which refers to structures lacking any mirror symmetry planes, is ubiquitous in nature, ranging from molecules and polymers to crystals. It is of great importance in biological and medical sciences as most biomolecules—the building blocks of life such as DNA—are chiral. Switching the handedness of chiral molecules under external stimuli has been found in various natural materials, such as organic molecules, sol-gel and even solid-state systems [1] , [2] , [3] , [4] , [5] , [6] . It is also particularly important in the study of stereochemistry and biology, as molecules with the same constituent atoms but different spatial configurations can result in significantly different physiological responses. Chirality of natural materials can be switched structurally by various means, such as photoexcitation [1] , [2] , [3] , [4] , electron tunneling [7] , application of electric fields [8] and temperature control [9] . Photoinduced chirality switching is of particular interest because of the ease of addressability. The underlying mechanism of chirality switching in organic molecules or polymers is a molecular structural change induced by an external stimulus, as illustrated in Fig. 1 . Examples are the photoinduced switching through the trans-cis isomerization of azobenzene and its derivatives [10] , [11] , [12] . The structurally induced chirality switching modifies the optical responses of molecules where the circular dichroism (CD), or the relative absorption between left-handed (LH) and right-handed (RH) circularly polarized waves, is reversed ( Fig. 1 ). As chiral molecules interact differently with electromagnetic waves of LH and RH circular polarizations, chirality switching is of great significance in controlling the polarization states. However, the optical activity in natural materials is very weak, and therefore the effect of chirality switching is not conspicuous. 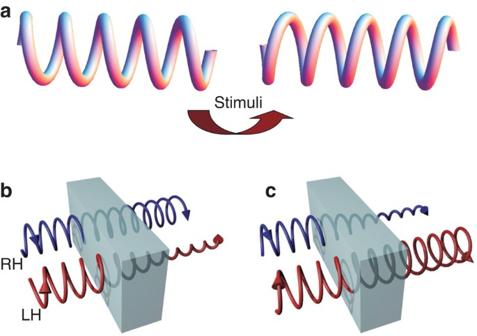Figure 1: The general principle of chirality switching in natural materials. (a) Schematic of a chiral molecule that lacks mirror symmetry in all directions. Under an external stimulus such as photoexcitation, temperature change or electric field, the chiral molecule undergoes a structural change to its mirror image, that is, the chirality is switched. (b) A material composed of the chiral molecules absorbs light more strongly for one circular polarization than the other. (c) After chirality switching, the chiral material reverses its responses to the two circular polarizations. Figure 1: The general principle of chirality switching in natural materials. ( a ) Schematic of a chiral molecule that lacks mirror symmetry in all directions. Under an external stimulus such as photoexcitation, temperature change or electric field, the chiral molecule undergoes a structural change to its mirror image, that is, the chirality is switched. ( b ) A material composed of the chiral molecules absorbs light more strongly for one circular polarization than the other. ( c ) After chirality switching, the chiral material reverses its responses to the two circular polarizations. Full size image Metamaterials are a new class of custom-designed composites with deep subwavelength building blocks, called metamolecules. Recent progress in metamaterials has led to the realization of gigantic optical activity that is several orders of magnitude stronger than that of natural materials [13] , [14] , [15] , [16] . However, the handedness of those chiral metamolecules was fixed once fabricated and could not be reconfigured in real-time. The concept of stereochemistry has been recently introduced to metamaterials; the change in the spatial configuration in metamolecules induces dramatic change in their optical properties [17] , [18] . A straight translation of chirality switching from organic molecules to metamolecules would be a structural reconfiguration of the metamolecule in response to an external stimulus. However, this would require a dynamically tunable mechanical system that entails great manufacturing complexity. Although mechanically tunable planar metamaterials have been demonstrated [19] , [20] , [21] , the structural tuning or twisting of three-dimensional complex chiral metamolecules still faces significant challenges, not to mention the slow switching speed that is generally intrinsic to mechanical systems. In this work, we show that, through designing a delicate artificial chiral metamolecule incorporated with a photoactive medium, we are able to transfer the concept of 'handedness switching' from organic chemistry to metamaterials without introducing any structural change, in stark contrast to the case of organic chiral molecules. We design optically switchable chiral terahertz metamaterials and experimentally observe handedness switching in the forms of reversed CD and reversed optical rotatory dispersion (ORD). It should be noted that the chirality (handedness) switching is a different process from the optically induced chirality in metamaterials previously demonstrated, where the chirality of a metamaterial was merely switched between on and off, but not reversed [22] . Benefitting from the strong switching effect in comparison to natural materials, the handedness-switching metamaterials may find important applications in terahertz technologies, ranging from vibrational CD for identification of the chirality and structures of organic molecules, to the precise non-contact Hall measurement. Experiment The terahertz chiral metamolecules are fabricated on top of a silicon-on-sapphire substrate (see Methods ). As shown in Fig. 2a,b , the structures are arranged in a fourfold rotational symmetry, such that the eigenmodes of the light propagating along normal incidence are circularly polarized. The unit cell has a lateral dimension of 50 μm, which is much less than the resonant wavelength of a few hundred micrometres in the terahertz frequency range, qualifying the chiral artificial structure as a metamaterial. Under strong optical illumination with photon energy greater than the bandgap of silicon, the excitation of photocarriers turns the incorporated silicon pads from insulating to highly conducting state, switching optoelectronically the electromagnetic chirality. Similar approaches of incorporating semiconductors into subwavelength resonators have been used to actively manipulate the electromagnetic resonances of metamaterials by photoexcitation or electric bias [23] , [24] , [25] , [26] . 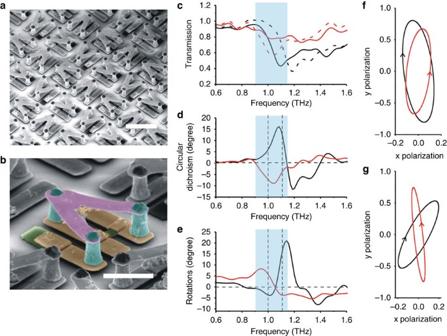Figure 2: Experimental demonstration of chiral switching metamaterials. (a,b) Scanning electron microscopy images of the fabricated metamaterial. The period of the metamaterial is 50 μm, which is far less than the wavelength of the terahertz waves. Scale bar in (a), 25 μm. In (b), the purple, blue and yellow colours represent the gold structures at different layers and the two silicon pads are shown in green. Scale bar, 10 μm. (c) The measured transmission spectra of LH (solid) and RH (dashed) circular polarizations, without (black) and with (red) photoexcitation. The shaded region represents the frequency range where the relative transmission amplitude between LH and RH polarization is reversed. (d) The CD spectrum (that is, ellipticity) and (e) the ORD derived from the measured transmission amplitude and phase spectra, without (black) and with (red) photoexcitation. In the shaded area, both the signs of CD and ORD are flipped, indicating the switching of handedness of the metamolecules. (f,g) The polarization states without (black) and with (red) photoexcitation for a linearly and vertically polarized incident terahertz beam transmitting through the chiral switching metamaterial at 1.0 and 1.1 THz, respectively. These two frequencies are also marked on the CD, and ORD spectra. At both frequencies, the polarization states turn from elliptical clockwise to elliptical anticlockwise under photoexcitation. Meanwhile, the major axis of the polarization ellipse is flipped from left to right at 1.0 THz, and from right to left at 1.1 THz. Figure 2: Experimental demonstration of chiral switching metamaterials. ( a , b ) Scanning electron microscopy images of the fabricated metamaterial. The period of the metamaterial is 50 μm, which is far less than the wavelength of the terahertz waves. Scale bar in ( a ), 25 μm. In ( b ), the purple, blue and yellow colours represent the gold structures at different layers and the two silicon pads are shown in green. Scale bar, 10 μm. ( c ) The measured transmission spectra of LH (solid) and RH (dashed) circular polarizations, without (black) and with (red) photoexcitation. The shaded region represents the frequency range where the relative transmission amplitude between LH and RH polarization is reversed. ( d ) The CD spectrum (that is, ellipticity) and ( e ) the ORD derived from the measured transmission amplitude and phase spectra, without (black) and with (red) photoexcitation. In the shaded area, both the signs of CD and ORD are flipped, indicating the switching of handedness of the metamolecules. ( f , g ) The polarization states without (black) and with (red) photoexcitation for a linearly and vertically polarized incident terahertz beam transmitting through the chiral switching metamaterial at 1.0 and 1.1 THz, respectively. These two frequencies are also marked on the CD, and ORD spectra. At both frequencies, the polarization states turn from elliptical clockwise to elliptical anticlockwise under photoexcitation. Meanwhile, the major axis of the polarization ellipse is flipped from left to right at 1.0 THz, and from right to left at 1.1 THz. Full size image The chirality switching in the above terahertz metamaterials was experimentally demonstrated through measurements using an optical-pump terahertz-probe (OPTP) spectroscopy system. The OPTP system provides 50-fs laser pulses with a centre wavelength of 800 nm and a repetition rate of 1 kHz to optically excite charge carriers in the silicon pads. Figure 2c shows the transmission spectra for the two circularly polarized terahertz waves. Without photoexcitation, the metamaterial strongly interacts with both LH and RH circular polarizations, but at different frequencies. This is demonstrated by the transmission dips at frequencies of 1.09 and 1.19 THz in the transmission spectra for LH (black solid) and RH (black dashed) circularly polarized waves, respectively. When illuminated by near-infrared laser pulses with fluence of about 1 mJ cm −2 , the resonance for LH polarization disappears and leaves a featureless transmission spectrum (red solid). Meanwhile, we observed a red-shifted resonance for RH polarization (red dashed) from 1.19 to 1.05 THz. As a result, the relative transmission amplitudes between the two circular polarizations are reversed in the frequency range between 0.9 and 1.14 THz, as marked by the shaded region. Within this frequency range, the RH polarization, which initially exhibited a higher transmission, yields a lower transmission than that of LH polarization with photoexcitation. CD and ORD are the two most commonly used techniques for characterizing the optical activity of chiral materials. CD refers to the difference between the transmission spectra of two circular polarizations, and therefore it is related to the ellipticity of the transmitted beam for a linearly polarized incident beam, and it can be calculated by θ =tan −1 [( E R − E L )/( E R + E L )]. Here E R(L) is the transmission amplitude for right (left)-handed circular polarizations. In contrast, ORD measures the polarization rotation angle arising from the transmission-phase difference between the two circular polarizations. As shown in Fig. 2d,e , within the shaded regions, both the signs of CD and ORD are indeed flipped. Interestingly, the ORD shows opposite switching behaviours at two frequency bands, from negative to positive between 0.9 and 1.05 THz, and from positive to negative between 1.05 and 1.19 THz. For an incident beam linearly polarized in the vertical direction, the representative polarization states of the transmitted wave are shown in Fig. 2f,g for two frequencies at 1.0 and 1.1 THz. At both frequencies, the polarization states of the transmitted wave are elliptical rotating clockwise when there is no photoexcitation (black). Under photoexcitation, the rotation is reversed to anticlockwise (red), and meanwhile, the polarization of the transmitted wave, that is, the orientation of the long axis of the polarization ellipses, is flipped from the left side of vertical axis (−3.6°) to the right side (5.7°) at 1.0 THz, and from the right side (13.8°) to the left side (−3.6°) at 1.1 THz. The flipped ORD, together with reversed CD, serve as direct evidences that the metamaterial exhibits a genuine chirality switching behaviour. The chirality switching effect of the demonstrated metamaterial is exceedingly strong, exhibiting a flipping of rotation angle in excess of 10° for a monolayer of metamolecules. Meanwhile, the switching is transient, and the sample will be restored to its original chiral state within milliseconds, determined by the lifetime of the photo-carriers in silicon. This relaxation time can be reduced by using photoactive materials with a shorter carrier lifetime. Numerical simulation We have performed full-wave simulations to validate the above chirality switching metamaterials using CST Microwave Studio. 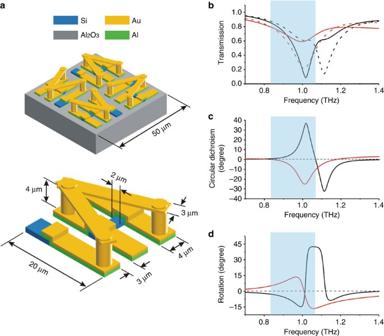Figure 3: Theoretical calculations on chiral switching metamaterials. (a) Schematic of the chirality switching metamaterial. The unit cell consists of four chiral resonators with fourfold rotational symmetry. The key geometrical parameters are labelled in the figure. (b) The transmission spectra of left-handed (solid) and right-handed (dashed) circular polarizations, without (black) and with (red) photoexcitation. The shaded region represents the frequency range where the relative transmission amplitude between LH and RH polarization is reversed. (c) The ellipticity calculated from the transmission spectra without (black solid) and with photoexcitation (red solid). In the shaded area the sign of circular dichroism is flipped. (d) The optical rotatory dispersion (ORD) without (black solid) and with optical pumping (red solid). These numerical results show good agreement with the experimental observations. Figure 3a shows the schematics of the unit cell of the metamaterial, which consists of four chiral resonators arranged with fourfold rotation symmetry. In the simulation, we have assumed a photo-conductivity of 5×10 4 S cm −1 for the optically irradiated silicon [25] . As shown in Fig. 3b , in the absence of photoexcitation, the transmission spectra of the LH (black solid curve) and RH (black dashed curve) polarizations exhibit a strong resonance feature, with a transmission dip <0.2, at 1.01 and 1.11 THz, respectively. These two resonances are consistent with the experimental results shown in Fig. 2 . With photoexcitation, the resonance for the LH polarization is dramatically weakened, and the resonance for the RH polarization is shifted to a lower frequency around 1.005 THz, that is, closely aligned with that for the LH polarization without photoexcitation, but slightly broadened and less pronounced because of the extra ohmic loss introduced by the optically doped silicon pad. The calculated CD and ORD spectra are shown in Fig. 3c,d . Reversed CD and ORD are simultaneously obtained in a broad frequency range from 0.84 to 1.07 THz, as marked by the shaded region. The simulation results are in reasonably good agreement with the experimental observations. Figure 3: Theoretical calculations on chiral switching metamaterials. ( a ) Schematic of the chirality switching metamaterial. The unit cell consists of four chiral resonators with fourfold rotational symmetry. The key geometrical parameters are labelled in the figure. ( b ) The transmission spectra of left-handed (solid) and right-handed (dashed) circular polarizations, without (black) and with (red) photoexcitation. The shaded region represents the frequency range where the relative transmission amplitude between LH and RH polarization is reversed. ( c ) The ellipticity calculated from the transmission spectra without (black solid) and with photoexcitation (red solid). In the shaded area the sign of circular dichroism is flipped. ( d ) The optical rotatory dispersion (ORD) without (black solid) and with optical pumping (red solid). These numerical results show good agreement with the experimental observations. Full size image The underlying mechanism responsible for the chirality switching in the terahertz metamaterial is illustrated schematically in Fig. 4 . We start from a chiral metamaterial design that has recently led to the demonstration of chirality-induced negative refractive index [14] . As shown by the equivalent inductor-capacitor (LC) circuit of the metamolecule in Fig. 4a , the metal loops function as inductors and the gap between the metal strips as capacitors of capacitance C . A single meta-atom exhibits a strong chirality at the LC resonance frequency, and consequently a positive or negative peak in CD spectrum depending on the chirality of the structure ( Fig. 4a ). When two chiral meta-atoms of the same shape but opposite chirality are assembled to form a metamolecule, the mirror symmetry is preserved, resulting in vanishing of optical activity. From a different point of view, the optical activity arising from these two meta-atoms of opposite chirality cancels out each other. 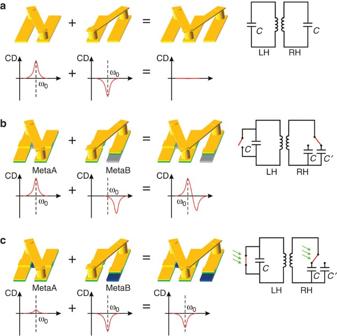Figure 4: Schematic design of chiral switching metamaterials illustrating the underlying mechanism. (a) A metamolecule consisting of two meta-atoms of opposite chirality. Each meta-atom is a three-dimensional gold split-ring resonator with its loop tilted relative to the gap, leading to the coupling between the electric and magnetic responses, and consequently, a strong chirality and large CD at its resonance frequency. When combined into a metamolecule, the optical activity arising from the two meta-atoms cancels each other out, resulting in a vanishing circular dichroism spectrum. The metamolecule can be represented by an equivalent circuit consisting of two LC resonators. (b) Silicon pads (gray) are incorporated to the metamolecule. The mirror symmetry is broken, and the metamolecule exhibits chirality at resonance frequencies. The silicon pads also function as the optoelectronic switches in the equivalent circuit. (c) With photoexcitation, photocarriers are generated in the silicon pads, leading to a switching of chirality in the form of reversed circular dichroism. Figure 4: Schematic design of chiral switching metamaterials illustrating the underlying mechanism. ( a ) A metamolecule consisting of two meta-atoms of opposite chirality. Each meta-atom is a three-dimensional gold split-ring resonator with its loop tilted relative to the gap, leading to the coupling between the electric and magnetic responses, and consequently, a strong chirality and large CD at its resonance frequency. When combined into a metamolecule, the optical activity arising from the two meta-atoms cancels each other out, resulting in a vanishing circular dichroism spectrum. The metamolecule can be represented by an equivalent circuit consisting of two LC resonators. ( b ) Silicon pads (gray) are incorporated to the metamolecule. The mirror symmetry is broken, and the metamolecule exhibits chirality at resonance frequencies. The silicon pads also function as the optoelectronic switches in the equivalent circuit. ( c ) With photoexcitation, photocarriers are generated in the silicon pads, leading to a switching of chirality in the form of reversed circular dichroism. Full size image We next introduce a silicon pad (gray) to each chiral meta-atom in the metamolecule, but at different locations, as shown in Fig. 4b . In one chiral atom (Meta-A), a silicon pad bridges the two base metal stripes, and in the other atom (Meta-B), a silicon pad replaces part of a base metal strip. The functions of silicon pads are twofold: they serve to break the mirror symmetry and induce chirality for the combined metamolecule, and function as optoelectronic switches to flip the chirality of the metamolecule under strong photoexcitation. For Meta-A, the insertion of the silicon bridge has very little effect on the resonance, as silicon has only slightly higher permittivity (11.7) than the sapphire substrate (10.5). Whereas the incorporation of silicon pad in Meta-B introduces a significant reduction of the capacitance of the equivalent LC circuit ( C ′< C ) due to the shortening of the metal strip, and therefore shifts the resonance towards a higher frequency. The combined structure—the metamolecule—exhibits a representative CD spectrum in Fig. 4b , where at the original resonance frequency ω 0 , the electromagnetic response of the metamolecule is dominated by Meta-A, as the resonance of Meta-B is shifted to a higher frequency. This explains the experiment observation shown in Fig. 2d (black curve). Under strong photoexcitation using near-infrared laser pulses with photon energy above the bandgap of silicon, the generation of high concentration of free charge carriers turns the originally nearly intrinsic silicon pads into conductors (denoted by the blue areas in Fig. 4c ). As shown by the equivalent circuit, this leads to an increase in the capacitance from C ′ to C , and consequently a red-shifting of resonance frequency of Meta-B to ω 0 . Meanwhile, the equivalent LC circuit for Meta-A is shortened due to photoexcitation. As a result, the CD is reversed, shown in Fig. 4c , as compared with the case without photoexcitation in Fig. 4b , which is in good agreement with the experimental observation of CD switching shown in Fig. 2d . Here we have proposed a general scheme to design active metamaterials, which can be switched between two opposite electromagnetic properties (in this case, left and right handedness). This scheme relies on the combination of two meta-atoms with opposite properties, one is functional but the other is inactive within the frequency range of interest. With suitable design, the two meta-atoms respond oppositely to an external stimulus, that is, the inactive one becoming functional and vice versa. This general design principle is not limited to handedness switching; it can also be applied to realize dynamic reversing of other electromagnetic functionalities. Sample fabrication The fabrication starts with a silicon-on-sapphire wafer. Silicon layer (600-nm thick) is patterned by photo-lithography (MA6, Karl Suss) and dry etched (PK-12 RIE, Plasma-Therm) to define the silicon pads ( Fig. 5a ). Aluminium (Al) is sputtered (300 nm; Auto 306, Edwards) onto the sample as an electrode for the subsequent electroplating process. On top of Al-covered silicon pads, 300-nm-thick gold pads are fabricated by photo-lithography, followed by electron beam evaporation (Solution, CHA Industries) and lift-off process ( Fig. 5b ). Five-micrometre-thick SU-8 (SU-8 3000, Microchem) is then coated and holes are patterned in the SU8 layer by photo-lithography and dry etching. Low current electroplating is performed to grow gold pillars in the holes ( Fig. 5c ). Gold bridges connecting the gold pillars are subsequently fabricated by photo-lithography and lift-off process ( Fig. 5d ). Finally, SU-8 and Al are removed by oxygen plasma etching and Al etchant (Type A, Transene Company), respectively, leading to the final structure shown in Fig. 2a,b . 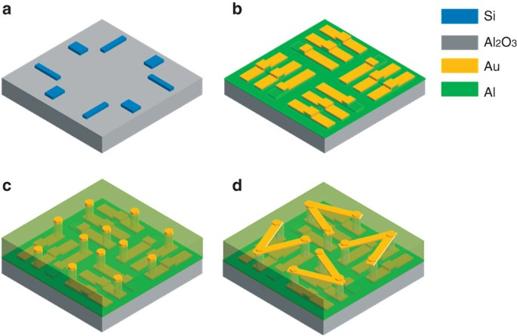Figure 5: Flowchart of the fabrication of the handedness switching metamaterials. (a) Patterning of silicon pads (blue) on top of the Al2O3substrate (gray) by photo-lithography and reactive ion etching. (b) Fabrication of gold pads on top of Al-coated silicon pads by a second photo-lithography followed by electron beam evaporation and lift-off process. (c) Coating of spin-on-glass and SU8 on the wafer, followed by patterning of holes in the SU8 by using photo-lithography and dry etching. Then, gold columns are created in the holes by electroplating. (d) Fabrication of gold bridges that connect the gold pillars by another photo-lithography process. Figure 5: Flowchart of the fabrication of the handedness switching metamaterials. ( a ) Patterning of silicon pads (blue) on top of the Al 2 O 3 substrate (gray) by photo-lithography and reactive ion etching. ( b ) Fabrication of gold pads on top of Al-coated silicon pads by a second photo-lithography followed by electron beam evaporation and lift-off process. ( c ) Coating of spin-on-glass and SU8 on the wafer, followed by patterning of holes in the SU8 by using photo-lithography and dry etching. Then, gold columns are created in the holes by electroplating. ( d ) Fabrication of gold bridges that connect the gold pillars by another photo-lithography process. Full size image Optical characterization We characterized the switchable chiral metamaterial using OPTP spectroscopy. The transmission of the linearly polarized terahertz pulses through the chiral metamaterial was measured in the time domain, with and without photoexcitation. Photoexcitation used near-infrared (~800 nm) laser pulses (50 fs) with a repetition rate of 1 kHz that illuminated the metamaterial sample a few picoseconds before the arrival of the terahertz pulses. The pump laser was focused down to a spot ~5 mm in diameter on the surface of the chiral sample, exciting electron-hole pairs across the 1.12 eV bandgap in all the silicon islands. To obtain the transmission coefficients of circularly polarized waves, that is, T + + , T − + , T + − and T − − , we measured four linear copolarization and cross-polarization transmission coefficients, T xx , T yx , T xy and T yy . Transmission coefficients of circularly polarized waves were then obtained from the linear measurements using the following equation: where the first and second subscripts refer to the incident and transmitted wave, + and − refer to the RH and LH circularly polarized waves, and x and y refer to the two linearly polarized waves with the electric field polarized along two orthogonal directions. How to cite this article: Zhang, S. et al . Photoinduced handedness switching in terahertz chiral metamolecules. Nat. Commun. 3:942 doi: 10.1038/ncomms1908 (2012).